Quantum oscillations of nitrogen atoms in uranium nitride The vibrational excitations of crystalline solids corresponding to acoustic or optic one-phonon modes appear as sharp features in measurements such as neutron spectroscopy. In contrast, many-phonon excitations generally produce a complicated, weak and featureless response. Here we present time-of-flight neutron scattering measurements for the binary solid uranium nitride, showing well-defined, equally spaced, high-energy vibrational modes in addition to the usual phonons. The spectrum is that of a single atom, isotropic quantum harmonic oscillator and characterizes independent motions of light nitrogen atoms, each found in an octahedral cage of heavy uranium atoms. This is an unexpected and beautiful experimental realization of one of the fundamental, exactly solvable problems in quantum mechanics. There are also practical implications, as the oscillator modes must be accounted for in the design of generation IV nuclear reactors that plan to use uranium nitride as a fuel. The spectrum of elementary excitations in materials is one of the core concepts in modern condensed matter physics. The archetypical example is the set of quantized lattice vibrations in crystalline solids, or phonons [1] . For crystals with more than one atom per unit cell, one expects both acoustic and optic phonon modes and if these are known, one can calculate the lattice contribution to fundamental properties such as the heat capacity. The vibrational spectrum at energies above those of the highest optic phonon mode is generally a complicated many phonon continuum that is often weak and featureless. In sharp contrast, for the binary solid uranium nitride (UN) [2] , [3] , [4] , [5] , where the nitrogen atoms are very light compared with the uranium atoms, our inelastic neutron-scattering measurements reveal that the high-energy spectrum is greatly simplified and consists of a set of equally-spaced, well-defined modes that can be measured to energies at least ten times as large as that of the optic phonon modes. This data is best explained by assuming that each nitrogen atom behaves as an independent quantum harmonic oscillator (QHO), and the nitrogen motion is therefore a rare experimental realization of an exactly soluble, three-dimensional model in quantum mechanics [6] . The binary uranium systems of the form UX (X = C, N, S, Se, Te, As, Sb) have relatively simple rocksalt crystal structures as illustrated in Fig. 1 . They have been extensively studied owing to their vast array of puzzling physical and magnetic properties [7] , including unusually high electronic-specific heats and drastic suppression of ordered magnetic moments. Among these systems, UN has received significant attention [8] , [9] , [10] , [11] , [12] recently owing to its potential use as a high-temperature nuclear fuel [13] , [14] , [15] . 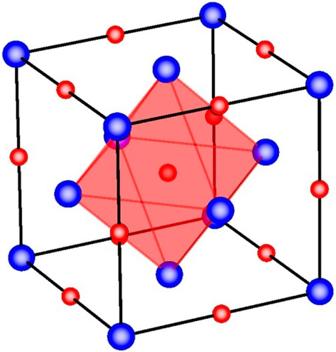Figure 1: Rocksalt crystal structure of uranium nitride. Each N atom (small red spheres) is centred in a regular octahedron of U atoms (large blue spheres). Figure 1: Rocksalt crystal structure of uranium nitride. Each N atom (small red spheres) is centred in a regular octahedron of U atoms (large blue spheres). Full size image The primary magnetic and lattice excitations of UN have been investigated previously via inelastic neutron scattering [2] , [3] , [16] . Despite these efforts, several intriguing open questions remain concerning the details of the experimental spectra. Since the initial measurements, significant advances have been made in inelastic neutron scattering using time-of-flight methods. Next-generation chopper spectrometers allow for measurements over much broader energy ( ω ) and momentum ( ) transfer ranges than were previously accessible, with both improved intensity and resolution. For these reasons, the excitations in UN were re-examined using the Fermi chopper spectrometers SEQUOIA [17] , [18] and ARCS [19] at the Spallation Neutron Source of Oak Ridge National Laboratory. In addition to the expected magnon and phonon modes, this investigation resulted in the unexpected discovery of a series of excitations spaced equally in energy by intervals of ~50 meV, and extending up to at least 500 meV. Conventional phonons To perform the measurements, the same UN crystal utilized by Jackman et al . 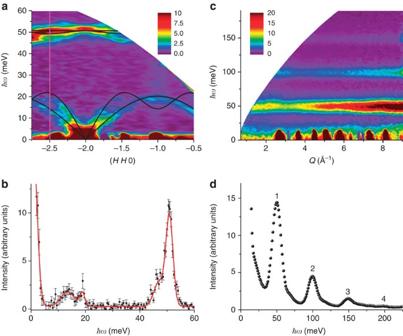Figure 2: Inelastic neutron scattering data from UN measured at SEQUOIA forT=5 K. (a) Colour intensity plot of the scattering withEi=80 meV. The vertical axisωdenotes the energy transfer, and the horizontal axis the wavevector transfer along high-symmetry direction (HH0). The integration ranges for the perpendicular directionsand (00L) were 0.2 reciprocal lattice units (r.l.u.). The data clearly shows the acoustic and optic one-phonon modes, and the black curves show fits of the phonon dispersion to the two force-constant model described elsewhere16. (b) A constantQ-cut taken along the vertical line inawith an integration range of 0.2 r.l.u. in the (HH0),and (00L) directions. The error bars represent one standard deviation from the expected signal, and the solid line depicts a fit to a superposition of Gaussian functions. (c) Colour intensity plot of theEi=250 meV data summed over all directions in reciprocal space, with the magnitude of the wavevector,Q, along the horizontal axis. Several modes are evident, evenly spaced in energy by ~50 meV intervals. As discussed in the text, these are attributed to QHO behaviour of the nitrogen atoms in UN. (d)Q-integrated data fromc, clearly showing the oscillator excitations. The error bars, representing one standard deviation from the expected signal, are smaller than the symbols. [2] was aligned with the ( HHL ) plane horizontal and cooled to a temperature T =5 K. Figure 2a shows representative results obtained at SEQUOIA using an incident neutron energy E i =80 meV for a typical symmetry direction in reciprocal space. A constant Q -cut through the data, at the position corresponding to the vertical line, is illustrated in Fig. 2b . The solid red curve is a fit to a superposition of Gaussian peaks at the mode positions. The measured phonon dispersion relations are consistent with earlier investigations [2] , [20] . The black lines in Fig. 2a are obtained from a fit of the data to a simplified model [16] that includes only nearest-neighbour U-N (65±2 N m −1 ) and U-U (50±4 N m −1 ) force constants. This model suffices for illustrative purposes, although more detailed models [2] , [8] , [9] , [10] , [21] , [22] give a closer match to the observed dispersion. Some of those models also include N-N force constants, although they are found to be negligibly small compared with their U-N and U-U counterparts. Figure 2: Inelastic neutron scattering data from UN measured at SEQUOIA for T =5 K. ( a ) Colour intensity plot of the scattering with E i =80 meV. The vertical axis ω denotes the energy transfer, and the horizontal axis the wavevector transfer along high-symmetry direction ( HH 0). The integration ranges for the perpendicular directions and (00 L ) were 0.2 reciprocal lattice units (r.l.u.). The data clearly shows the acoustic and optic one-phonon modes, and the black curves show fits of the phonon dispersion to the two force-constant model described elsewhere [16] . ( b ) A constant Q -cut taken along the vertical line in a with an integration range of 0.2 r.l.u. in the ( HH 0), and (00 L ) directions. The error bars represent one standard deviation from the expected signal, and the solid line depicts a fit to a superposition of Gaussian functions. ( c ) Colour intensity plot of the E i =250 meV data summed over all directions in reciprocal space, with the magnitude of the wavevector, Q , along the horizontal axis. Several modes are evident, evenly spaced in energy by ~50 meV intervals. As discussed in the text, these are attributed to QHO behaviour of the nitrogen atoms in UN. ( d ) Q -integrated data from c , clearly showing the oscillator excitations. The error bars, representing one standard deviation from the expected signal, are smaller than the symbols. Full size image Notably, the optic modes are well separated in energy from the acoustic modes and are weakly dispersive centred around ω ~50 meV [2] , [20] . Because of the large mass ratio M / m , where M and m are the masses of the U and N atoms, respectively, the eigenvectors of the modes are such that the U atom motions are largely reflected by the acoustic phonons and the optic modes correspond primarily to motions of the N atoms [16] . A weak column of magnetic scattering, previously observed by Holden et al . [3] , is also visible in Fig. 2a at the antiferromagnetic zone centre (−1 −1 0). High energy response The upper and lower panels in Fig. 2c,d show SEQUOIA data taken with E i =250 meV covering a larger range of energy transfer. The upper panel shows the data averaged over all measured crystal orientations and the lower panel is a plot of intensity versus energy transfer for this data summed over Q . The data is striking and reveals a series of essentially dispersionless excitations extending up in energy from the optic mode, and evenly spaced by ~50 meV intervals. The intensity of each mode increases with increasing momentum transfer over several Å −1 indicating that these excitations are vibrational as opposed to magnetic. These data were extended greatly in both energy and wavevector range by further measurements using the ARCS chopper spectrometer. The larger Q range of this instrument is provided by its wide-angle detector coverage up to 2 θ ~135°, whereas the maximum 2 θ for SEQUOIA is only ~60°. 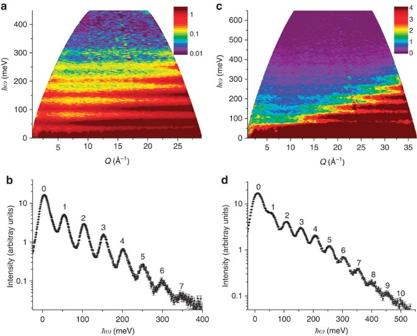Figure 3: Inelastic neutron scattering data from UN measured at ARCS forT=5 K. (a) Colour intensity plot of the scattering withEi=500 meV averaged over all measured crystal orientations. (b) The scattering inaintegrated over allQ, with the error bars representing one standard deviation from the expected signal. (c) Colour intensity plot of the scattering withEi=800 meV averaged over all measured crystal orientations. (d) The scattering incintegrated over allQ, with the error bars representing one standard deviation from the expected signal. Figure 3a,b show ARCS data with E i =500 meV plotted on a logarithmic intensity scale. Figure 3c,d show data from the same instrument with E i =800 meV; the upper panel c has intensity on a linear scale, whereas panel d is also on a logarithmic scale. A series of evenly spaced excitations is clearly visible up to the 10th order at an energy of 500 meV. The well-defined peaks in the orientationally averaged data imply that the modes are localized and isotropic, and the energy widths of these excitations were found to be roughly the same for all orders of n . Figure 3: Inelastic neutron scattering data from UN measured at ARCS for T =5 K. ( a ) Colour intensity plot of the scattering with E i =500 meV averaged over all measured crystal orientations. ( b ) The scattering in a integrated over all Q , with the error bars representing one standard deviation from the expected signal. ( c ) Colour intensity plot of the scattering with E i =800 meV averaged over all measured crystal orientations. ( d ) The scattering in c integrated over all Q , with the error bars representing one standard deviation from the expected signal. Full size image QHO model Some enhanced response at an energy corresponding to twice that of the optic phonon was observed in previous neutron scattering studies of UN and attributed to two-phonon processes [16] . However, the observation of such an extended series of equally spaced and well-defined modes is unprecedented. The most obvious system exhibiting a spectrum consisting of equally spaced modes is the QHO. Here one can postulate that the extremely light mass of the N atom relative to the U atom leads to a situation where high-frequency vibrations in the crystal essentially consist of motions of individual N atoms in a very isotropic and harmonic potential arising from a surrounding regular octahedron of U atoms. Each N atom is then a nearly ideal realization of the QHO in three dimensions, with a fundamental frequency corresponding to an energy ω o ≈50 meV, equivalent to a temperature of 580 K. The QHO is one of the simplest and best understood theoretical models in quantum mechanics [6] , and serves as the foundation for understanding diverse phenomena such as the vibrational modes of molecules, the motion of atoms in a lattice and the theory of heat capacity. We show below that the QHO model can quantitatively describe the high-energy vibrational features observed in the UN data. The neutron-scattering signal expected from the QHO is well known [23] . The dynamical response for k B T ≪ ω o can be written as: where the contribution to the intensity arising from the n th oscillator excitation is given by: The argument of the exponent resembles a Debye–Waller factor and reflects the zero-point motion of the oscillator. It is interesting to note that the intensity maximum for each mode occurs at the Q position corresponding to the recoil scattering for a free particle of mass m (see Supplementary Discussion Section A and Supplementary Fig. S1 for further details). Equation (2) reflects the intensity expected for a single inelastic scattering event. As the modes are evenly spaced, in a real experiment multiple scattering events in any combination of elastic and inelastic scattering will also result in intensity at the positions of the modes. Hence, any comparison of the QHO theory to the data must account for the intensity arising from multiple scattering in some fashion. As a first approximation, the measured data for UN was compared with the QHO model by fitting constant energy cuts (20 meV integration range) corresponding to the n =1–7 modes for both E i =500 meV and 800 meV data to the following functional form: Here the multiple scattering contribution to the observed intensity at each mode position is assumed to be a constant B n independent of momentum Q : this is the simplest possible assumption. The B n term and the associated multiple scattering are discussed in more detail in Supplementary Discussion Section B and Supplementary Fig. S2 . 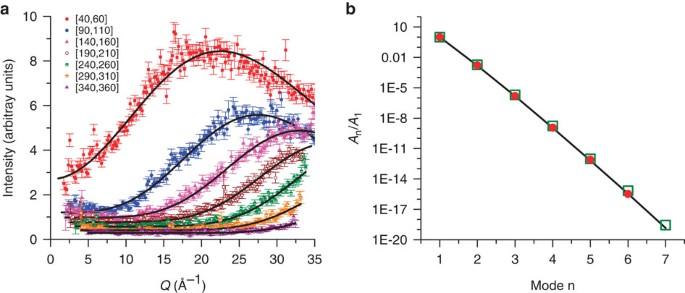Figure 4: Fitting results and analysis of the UN oscillator modes. (a) TheQ-dependence of the intensity for then=1–7 oscillator modes withEi=800 meV. The error bars represent one standard deviation from the expected signal, and the legend indicates ranges of integration over energy transfer in meV. The solid lines are fits to the QHO model as described in the text. (b) TheAncoefficients for then=1–7 modes normalized by the values ofA1. The coefficients are extracted from fits to theEi=500 meV (solid red circles) and 800 meV (open green squares) ARCS data sets, and the error bars, representing one standard deviation, are smaller than the size of the symbols. The solid line is the prediction of the QHO model withωo=50 meV andmcorresponding to the mass of a nitrogen atom. The ratio is plotted on a logarithmic scale and spans almost 20 orders of magnitude. Figure 4a shows the Q dependence of the seven lowest oscillator modes for the E i =800 meV data with solid lines indicating the corresponding fits to equation (3). The fits are excellent over the entire range of measured data and this is also true for the E i =500 meV data (not shown). Figure 4b plots the ratios of the fitted parameters A n / A 1 for both data sets. The solid curve indicates the prediction of the QHO model for a nitrogen atom with ω o =50 meV, with the non-integer n values interpolated by using Γ( n +1) to calculate n !. The values obtained from the data agree very well with the model over nearly 20 orders of magnitude. The maximum relative deviation for any one ratio is within a factor of two for the E i =800 meV data and within 20% for the E i =500 meV data. Given the large range of values covered and the simple assumption made for the multiple scattering, this is strong confirmation that the QHO picture applies to the nitrogen atoms in the uranium lattice. Figure 4: Fitting results and analysis of the UN oscillator modes. ( a ) The Q -dependence of the intensity for the n =1–7 oscillator modes with E i =800 meV. The error bars represent one standard deviation from the expected signal, and the legend indicates ranges of integration over energy transfer in meV. The solid lines are fits to the QHO model as described in the text. ( b ) The A n coefficients for the n =1–7 modes normalized by the values of A 1 . The coefficients are extracted from fits to the E i =500 meV (solid red circles) and 800 meV (open green squares) ARCS data sets, and the error bars, representing one standard deviation, are smaller than the size of the symbols. The solid line is the prediction of the QHO model with ω o =50 meV and m corresponding to the mass of a nitrogen atom. The ratio is plotted on a logarithmic scale and spans almost 20 orders of magnitude. Full size image The parameter C is related to the zero-point energy of the oscillator. For a nitrogen atom in a harmonic potential corresponding to ω o =50 meV, the calculated value of C is 0.003 Å 2 . The mean value of C determined from all modes at both incident energies was found to be 0.00275(10) Å 2 ; this is very close to the calculated value. As a further check, the data for each E i was analysed using a global fit (see Supplementary Discussion Section B and Supplementary Fig. S3 ) obtaining values for C of 0.00276(2) Å 2 and 0.00264(2) Å 2 for the E i =500 meV and 800 meV data sets, respectively, also in good agreement with expectations. The slight discrepancies between the fitted and calculated C values may be due to the simple assumption made for the multiple scattering. Binary solid model extension Clearly, the QHO model gives an outstanding description of the data. It should be noted that a calculation of the multiphonon scattering for a single frequency, perfectly dispersionless Einstein model leads to a result that is equivalent to the QHO model [24] . However, the oscillator picture is a simpler and more physically reasonable description for the localized vibrations of N atoms in UN, particularly when one considers that it is not an ideal Einstein solid: the crystalline environment and acoustic modes also affect the scattering. Detailed theoretical predictions exist for the response of a binary harmonic solid consisting of a lattice of diatomic molecules with a light atom of mass m bound to a heavier atom of mass M [25] . In the limit m ≪ M , appropriate for UN, the finite mass of the U atoms can be accounted for approximately by replacing the delta function in equation (2) with a Gaussian: This modification suggests that the oscillator modes should be broadened to a width σ and the position of the n th mode shifted by the uranium recoil to . For UN, it is not possible to associate a specific N atom with an individual U atom, nevertheless it is still reasonable to compare the data with the binary solid model. To assess how well this model describes the present data, constant Q -cuts (2 Å −1 integration range) from the ARCS E i =500 meV measurement were fit to a superposition of several Gaussian functions (see Supplementary Fig. S4 for a representative fit). The net result of the fitting shows that the modes have an average intrinsic full-width half-maximum of 26 meV with no systematic behaviour evident as a function of Q or n (see Supplementary Table S1 and Supplementary Fig. S5 ). The magnitude of the broadening is in agreement with the prediction of the binary solid model [25] that the intrinsic energy width of the n >1 peaks should be of the same order as the bandwidth of the acoustic phonon modes. Inspection of Fig. 2a shows this width to be around 20 meV. Except for a possible small effect on the n =1 mode, the fitting does not reveal a measurable shift of the mode energies as a function of Q . Multiple scattering contributions at the mode positions may mask any shift at higher Q . More details of the binary solid model extension are provided in Supplementary Discussion Section C . Local potential of the nitrogen atoms To investigate why the isotropic QHO description is so appropriate for UN, density functional theory (DFT) has been used to calculate the potential energy of the nitrogen atoms relative to their equilibrium positions for displacements along major crystallographic directions. Although DFT often fails to give the true ground state for correlated materials, in fact it has been shown to give a good description of the electronic energies in UN [10] . Moreover, DFT gives highly reliable values for relative energy differences of displaced atoms independent of the precise ground state. The DFT results shown in Fig. 5 verify that the potential is harmonic over a wide energy range, certainly for E <1 eV. At the same time, in this range, the potential energy along different directions is isotropic to within 2%. The ab-initio calculations predict an energy spacing for the oscillator modes of 50 meV, corresponding very well to the spacing of the excitations observed in the neutron-scattering measurements. 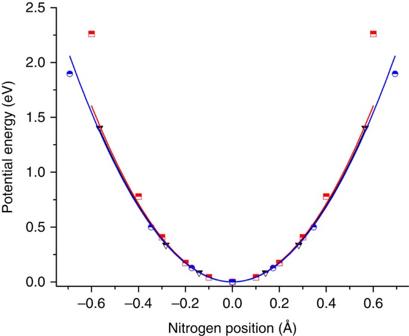Figure 5: DFT calculated potential energy of the N atoms in the system UN. The potential energy is shown for atomic displacements relative to the equilibrium position along the [100] (red squares), [110] (black triangles) and [111] (blue circles) directions. The solid lines are fits of the calculated small displacement limit values to parabolic (that is harmonic) potentials. The potential energy is very isotropic and harmonic over a wide range. Deviations are visible above 1 eV, especially along the [100] direction. Figure 5: DFT calculated potential energy of the N atoms in the system UN. The potential energy is shown for atomic displacements relative to the equilibrium position along the [100] (red squares), [110] (black triangles) and [111] (blue circles) directions. The solid lines are fits of the calculated small displacement limit values to parabolic (that is harmonic) potentials. The potential energy is very isotropic and harmonic over a wide range. Deviations are visible above 1 eV, especially along the [100] direction. Full size image The QHO behaviour observed here should be visible in many materials where the constituent atoms have greatly different masses. It is also important that there be weak interactions between light atoms sitting in a very harmonic potential. Possible harmonic oscillator behaviour has long been sought and investigated in metallic hydrides, especially for zirconium and titanium systems [26] , [27] , [28] , [29] , [30] , [31] . However, the potentials at the hydrogen sites generally show significant anisotropy or anharmonic effects [32] , [33] . These features manifest themselves as fine structure and uneven spacing in the hydrogen vibrational modes, and they arise from H–H interactions, crystalline anisotropy and low potential barriers to hopping of the protons. In sharp contrast, the potential at the nitrogen sites of UN is very harmonic and isotropic, leading to evenly spaced nitrogen vibrational modes exhibiting no fine structure within the instrumental energy resolution. To the best of our knowledge, each nitrogen atom in UN is a unique manifestation of a single-atom QHO. The scattering of neutrons from the oscillator modes may be an important factor in the consideration of UN as a nuclear fuel material. UN has several desirable characteristics for this application, including excellent thermal conductivity and a high melting temperature. For that reason, it is currently under intense consideration for use in proposed Generation IV nuclear reactors [13] , [14] , [15] , [34] , which operate at high temperatures (500–1,000 °C), allowing for improved efficiency in the conversion of heat to electricity. Nuclear reactor designs require a detailed knowledge of the neutron cross-sections and thermal behaviour of the constituent atoms composing the nuclear fuel. Fermi [35] showed that harmonic oscillations of protons in metals have a significant measurable effect on total neutron cross-sections. In addition to affecting the total cross-section, the oscillator modes in UN could also impact operation via self-moderation of neutrons. The modes will be thermally populated at the proposed Generation IV-operating temperatures and it is necessary to understand if there will be any impact on the thermal conductivity. Given the strong scattering processes shown in the present work, it is clear that the oscillator excitations must be accounted for properly in any detailed Generation IV designs. Neutron scattering For the neutron scattering experiments, the UN single crystal was sealed in an ultrathin Al sample can [36] with He exchange gas and cooled to ~5 K in a closed cycle He refrigerator. For the SEQUOIA [18] measurements, a Fermi chopper with a slit spacing of 3.6 mm and a radius of curvature of 1.53 m was spun at 300 Hz and 360 Hz for E i =80 meV and 250 meV, respectively, yielding FWHM energy resolutions of 4% and 6% of E i at the elastic line. The data was accumulated by combining measurements taken with several different incident neutron directions in the [ HHL ] plane. The data from ARCS was obtained using a chopper with an identical radius of curvature and outer dimensions to the SEQUOIA Fermi chopper described above, but with a slit spacing of 0.5 mm. The chopper was spun at 480 Hz ( E i =500 meV) or 600 Hz for ( E i =800 meV) to yield a FWHM energy resolution of 3.5% of E i at the elastic line. The sample was rotated continuously between the [ HH 0] and [00 L ] directions during data collection. In all measurements, the data was normalized to account for variations of the detector response and solid angle coverage with a vanadium standard. This procedure enabled an accurate determination of the orientationally averaged scattering response. The collection of neutron events is a counting process, therefore we used Poisson statistics for computing uncertainties. Density functional theory The electronic structure within the DFT was obtained using the Quantum ESPRESSO package [37] . The calculation was performed using a plane-wave basis set and ultrasoft pseudopotential [38] in a RKKJ scheme [39] . The uranium pseudopotential was obtained from an ionized electronic configuration 6 p 6 6 d 1 5 f 3 7 s 1 with cut-off radii equal to 3.5 atomic units (a.u. ), 1.7, 2.6 and 1.6 a.u. for s , p , d and f angular momentum. The electronic levels deviate from the all-electron ones by less than 0.1 meV. We used the Perdew, Burke and Ernzerhof [40] exchange-correlation functional. The Brillouin zone (BZ) summations were carried out over a 4×4×4 BZ k-points grid for a supercell containing 64 atoms. The electronic smearing with a width of 0.02 Ry was applied according to the Methfessel–Paxton method. The plane wave energy and charge density cut-offs were 73 Ry and 1054 Ry, respectively, corresponding to a calculation accuracy of 0.2 mRy per atom. The nitrogen atom potential was obtained from the total energy modification of a 2×2×2 supercell when one nitrogen atom was shifted from the equilibrium position in the [100], [110] or [111] directions and the remaining atoms were held fixed in their equilibrium positions. How to cite this article: Aczel A. A. et al . Quantum oscillations of nitrogen atoms in uranium nitride. Nat. Commun. 3:1124 doi: 10.1038/ncomms2117 (2012).